Chemically programmed self-sorting of gelator networks Controlling the order and spatial distribution of self-assembly in multicomponent supramolecular systems could underpin exciting new functional materials, but it is extremely challenging. When a solution of different components self-assembles, the molecules can either coassemble, or self-sort, where a preference for like-like intermolecular interactions results in coexisting, homomolecular assemblies. A challenge is to produce generic and controlled ‘one-pot’ fabrication methods to form separate ordered assemblies from ‘cocktails’ of two or more self-assembling species, which might have relatively similar molecular structures and chemistry. Self-sorting in supramolecular gel phases is hence rare. Here we report the first example of the pH-controlled self-sorting of gelators to form self-assembled networks in water. Uniquely, the order of assembly can be predefined. The assembly of each component is preprogrammed by the p K a of the gelator. This pH-programming method will enable higher level, complex structures to be formed that cannot be accessed by simple thermal gelation. When self-assembly occurs in a solution of two different molecules, several different outcomes are possible. The molecules may coassemble, either randomly or specifically or, alternatively, the molecules may segregate and ‘self-sort’ [1] , [2] , [3] . In a self-sorting system, the molecules discriminate between self and non-self such that pure assemblies of one molecule coexist with pure assemblies of the other ( Fig. 1 ). 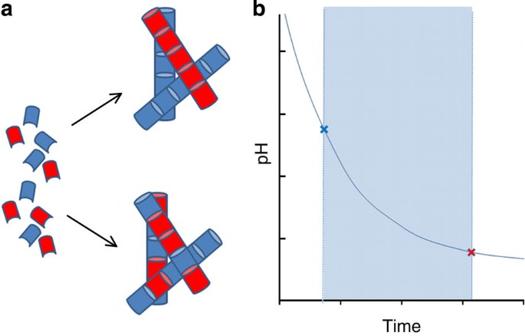Figure 1: Schematic of self-sorting. (a) Two molecules can either randomly coassembly (bottom) or self-sort (top) to form aggregated structures. (b) If two molecules have different pKavalues, then a slow pH decrease will lead to the pKaof one molecule being reached first (blue cross). Assembly occurs before the pKaof the second molecule (red cross) is reached. This leads to sequential assembly. Figure 1: Schematic of self-sorting. ( a ) Two molecules can either randomly coassembly (bottom) or self-sort (top) to form aggregated structures. ( b ) If two molecules have different p K a values, then a slow pH decrease will lead to the p K a of one molecule being reached first (blue cross). Assembly occurs before the p K a of the second molecule (red cross) is reached. This leads to sequential assembly. Full size image This method is being applied to the preparation of more complex, higher-order, self-sorted systems for applications such as catalysis [4] , as well as in the formation of p-n bulk heterojunctions via the assembly of two components into independent fibres of electron rich and electron poor gelators [5] . However, designing self-sorting systems is difficult and requires either known specific interactions or the choice of molecules where the self-association specificities are very different, thus limiting the potential for the preprogrammed assembly of a wide range of functional architectures. Self-sorting in supramolecular gel phases is a rare phenomenon and, at present, always achieved via thermally induced gelation [6] , [7] , [8] , [9] , [10] , [11] , [12] . Typically, a solution containing the two types of gelator molecule is heated above the temperature required to dissolve both completely. On cooling, one molecule assembles at a higher temperature than the other, which can result in a self-sorted network. Formation of such a self-sorted network is often inferred from visual differences between self-assembled structures as imaged by scanning electron microscopy (SEM), atomic force microscopy or transmission electron microscopy (TEM) [6] , [7] , [8] . For example, Shinkai and colleagues [5] have demonstrated that a bulk heterojunction can be formed via the thermal self-sorting of two specific gelators that self-assemble to form fibres, with the junctions between fibres giving rise to the heterojunction. These studies have concentrated on organogels. Extending this self-sorting concept to hydrogels represents a more difficult challenge because competitive hydrogen-bonding with water molecules can render many means of inducing self-sorting ineffective. The ability to regulate self-sorting behaviour by external stimuli was highlighted recently as a major challenge [1] . Thermally induced self-sorting, however, is difficult to predict and to design, as there is little correlation between the molecular structure and the assembly temperatures. A more powerful approach would be a chemically programmed method whereby the order of gelation could be controlled by a predictable ‘molecular trigger’, such that complex structures can be built in a targeted manner. We recently described the self-assembly of a range of naphthalene-functionalized dipeptide hydrogelators ( Fig. 2a ) 13,14 [13] , [14] . In these cases, gelation is triggered by a decrease in pH from 10.5 to just below the apparent p K a of the terminal carboxylic acid. The apparent p K a of these dipeptides is linked to the overall hydrophobicity of the molecule [14] , providing an easily variable ‘molecular gelation trigger’ that can be controlled by careful design of the gelator molecule. These molecules form gels by assembly into one-dimensional fibres, which entangle at suitable concentrations causing gelation of the host solvent. The self-assembly of these molecules starts to occur at the apparent p K a (ref. 13 ), such that the pH at which gels form correlates well with the apparent p K a . This allows the pH at which self-assembly occurs to be predicted from a simple parameter describing the molecular structure. To form the gels, we exploited the hydrolysis of glucono-δ-lactone (GdL) to gluconic acid ( Fig. 2b ) 13,15,16 [13] , [15] , [16] . The hydrolysis allows a slow, uniform pH change in the system. A controlled pH decrease has two key benefits over mineral acids: (i) the hydrolysis and self-assembly of these gelators occurs over the timescale of hours and (ii) more homogeneous gels result [16] . Here we show that coupling the predictable apparent p K a of these molecules with the slow hydrolysis of GdL allows the predictable formation of hydrogels and, unprecedentedly, that mixed gelators undergo self-sorting via this route ( Fig. 1a (top) ). We note that mixed Fmoc-dipeptide-based gelling systems have been described previously [17] , [18] , [19] , [20] and that Van Esch has shown that self-sorting between a hydrogelator and a surfactant can take place in water [21] , [22] . However, in the case of mixed dipeptide gelators, these were assumed to coassemble to form fibres randomly containing both gelators. 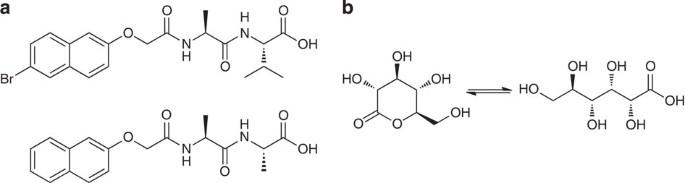Figure 2: Chemical structures. (a) Structures of gelators1(top) and2(bottom); (b) Hydrolysis of GdL to gluconic acid. Figure 2: Chemical structures. ( a ) Structures of gelators 1 (top) and 2 (bottom); ( b ) Hydrolysis of GdL to gluconic acid. Full size image NMR demonstration of sequential assembly We demonstrate self-sorting with two gelators ( 1 and 2 , Fig. 2 ); we have described the gelation process of 1 in detail previously [13] and shown that 2 forms gels [14] , but can crystallise under certain conditions [23] . Both 1 and 2 form self-supporting hydrogels in single-component systems (rheological data is shown in Supplementary Fig. S1 ) [13] , [14] . At concentrations of 5.0 mg ml −1 in D 2 O, 1 has an apparent p K a of 5.9, while 2 has an apparent p K a of 5.1. On the basis of this difference, we hypothesized that, in a mixed system, 1 should assemble at a higher pH than 2 ( Fig. 1b ). We note here that a range of p K a values is possible in molecules of this type [14] , [23] , and hence this approach offers the potential of ‘dialling in’ assembly at specific pH values to create complex, multicomponent structures. Mixing stock solutions of gelators 1 and 2 at high pH (pH 10.5; 5 mg ml −1 for both 1 and 2 ) results in a free-flowing solution without the need for heating. We initially probed the assembly that accompanies a reduction in pH by using solution NMR. This method has previously been used to follow thermally self-sorting gels [6] . When self-assembly leads to high molecular weight, solid-like fibres, the structures become NMR-invisible [24] , [25] . It is immediately apparent that, after addition of GdL, 1 became NMR-invisible before 2 , which is strongly indicative of sequential gelation ( Fig. 3a ). The hydrolysis of GdL is highly reproducible; hence knowing the starting pH, the temperature, and the peptide concentrations, the pH decrease can be measured and, therefore, the pH determined at any specific time (see for example Supplementary Fig. S2 ). Using this method, we were able to measure the pH at which both 1 and 2 start to become NMR-invisible. Example data for a GdL concentration of 12.6 mg ml −1 is shown in Fig. 3a (final pH=4.3). In line with our hypothesis, the disappearance of NMR signals arising from the dipeptides in solution correlates with the points at which the pH was slightly below the p K a of each component [14] . At this GdL concentration, 1 assembles completely before 2 begins to assemble, as shown by the complete loss of signal from 1 before any disappearance of 2 . These data, therefore, demonstrates unequivocally the consecutive assembly of the gelators, rather than simultaneous coassembly. A transparent gel is again formed from this mixed system (rheological data shown in Supplementary Fig. S1 ). The rheological data show that G′ is at least an order of magnitude greater than G″ as expected for a true gel. Also both G′ and G″ are frequency independent as expected for a gel formed from a fibrillar network. 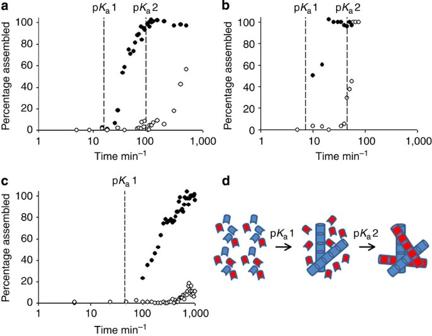Figure 3: NMR data show sequential assembly. Data derived from integration of NMR data showing that dipeptide1(·) assembles first, followed by dipeptide2(○). Assembly occurs at a pH slightly below the pKaof each component (shown by the vertical dotted lines). (a) Data for 12.6 mg ml−1GdL; (b) data for 43 mg ml−1GdL; (c) data for 5.4 mg ml−1GdL. In all cases, the initial solutions were identical; (d) shows a schematic cartoon of the process. Figure 3: NMR data show sequential assembly. Data derived from integration of NMR data showing that dipeptide 1 (·) assembles first, followed by dipeptide 2 ( ○ ). Assembly occurs at a pH slightly below the p K a of each component (shown by the vertical dotted lines). ( a ) Data for 12.6 mg ml −1 GdL; ( b ) data for 43 mg ml −1 GdL; ( c ) data for 5.4 mg ml −1 GdL. In all cases, the initial solutions were identical; ( d ) shows a schematic cartoon of the process. Full size image Exquisite control over the self-sorting process is achievable by careful control of the GdL concentration and, hence, control of both the rate of pH change and the final pH. The assembly of 1 before 2 occurred irrespective of the rate of pH change (as varied by altering the initial concentration of GdL). By adjusting the amount of GdL added, it was possible to assemble 1 alone in a mixture of 1 and 2 ( Fig. 3c : 5.4 mg ml −1 GdL, final pH=5.6). At increased concentrations of GdL, both 1 and 2 assembled ( Fig. 3b : 43 mg ml −1 GdL, final pH =3.3), but at an increased rate as compared with the data in Fig. 3a . A schematic of self-sorting assembly process is shown in Fig. 3d . The pH data is shown in Supplementary Fig. S2 and Supplementary Table S1 . Microscopy of sequentially assembled systems Although the NMR data is evidence that the assembly process is sequential for these two gelators, it is not unequivocal proof of self-sorting—that is, that separate, unique structures are formed without, for example, scrambling or rearrangement of the gelators once both molecules have sequentially self-assembled. Unlike observations for other self-sorted systems [6] , [7] , we were unable to categorically prove self-sorting using microscopy (TEM, Fig. 4 or SEM, Supplementary Fig. S3 ). Representative TEM images of 1 and 2 are shown in Fig. 4a , respectively. 1 showed the presence of single fibrils of 17.3 nm (±1.97 nm), bilaterally associated fibrils with diameters of 22.9 nm (±0.90 nm), and double-striated fibrils with diameters of 26.9 nm (±1.23 nm). The morphologies observed here are comparable with our previous reports on 1 (ref. 13 ). Gels of 2 contained predominantly single fibrils with a diameter of 8.9 nm (±1.16 nm) and also bilaterally associated fibrils of 16.1 nm (±0.86 nm). The diameter and degrees of lateral association are the best descriptors of the morphologies of these systems and thus this was assessed in the mixed system. A representative image of the mixed system is shown in Fig. 4c , showing single filaments with a diameter of 13.3 nm (±1.46 nm), bilaterally associated filaments with a diameter of 19.4 nm (±1.95 nm) and double-striated fibrils with diameters of 24.9 nm (±1.44 nm). 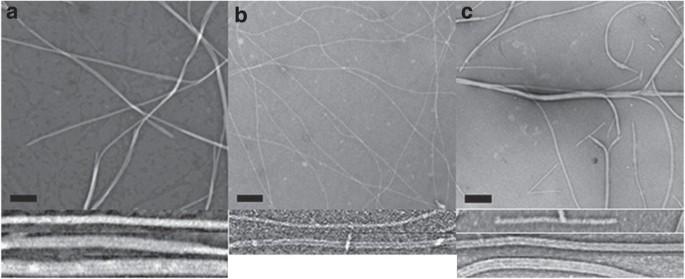Figure 4: Microscopy of mixed and single systems. TEM of a gel of (a)1alone; (b)2alone and (c) mixed1and2. Scale bars represent 200 nm. The corresponding insets show expansions (not to scale) highlighting the morphologies of each system:1contains single filaments, bilaterally associated filaments and thicker fibrils with double striations.2contains predominantly single, and some bilaterally associated filaments. The mixed system has morphologies consistent with1. Figure 4: Microscopy of mixed and single systems. TEM of a gel of ( a ) 1 alone; ( b ) 2 alone and ( c ) mixed 1 and 2 . Scale bars represent 200 nm. The corresponding insets show expansions (not to scale) highlighting the morphologies of each system: 1 contains single filaments, bilaterally associated filaments and thicker fibrils with double striations. 2 contains predominantly single, and some bilaterally associated filaments. The mixed system has morphologies consistent with 1 . Full size image To thoroughly assess fibril morphology, 127–283 unique measurements of fibril diameters were made for the single and mixed system ( Supplementary Fig. S4 ); the mixed system was found to contain filaments characteristic of 1 although with some perturbation in size. The presence of fibrils characteristic of 1 is corroborated by visual inspection of the micrographs ( Fig. 4a–c insets). The observation of filaments of 1 in the mixed solution ( Fig. 4c ) is strongly suggestive of self-sorting, though alone is not sufficient to unambiguously show self-sorting at this macroscopic level. Small-Angle Neutron Scattering indicates self-sorting To further distinguish coassembly from self-sorting, small-angle neutron scattering (SANS) was performed to probe the self-sorting at the nanoscale. Given the finite Q range of the instrument used (1–100 nm), the fitting is most sensitive to the cross-sectional nature of the filament, hence SANS is in principle a good tool to evaluate gels with self-sorted fibres of different diameters. To fit the data, which exhibits a smooth transition in Q dependence over the length scale probed on the instrument, Fig. 5 , we used the Kholodenko-Dirac worm-like chain model. The best fit to the data for 1 using this model (solid line) was for a core-shell structure with a core radius ( R core ) of 5.2 nm and an outer radius ( R outer ) of 8.8 nm, implying a shell thickness of 3.6 nm. 2 alone exhibited very different scattering to 1 ,with the data fitting best to the simpler solid worm-like structure, with a radius of 2.6 nm. In both cases, the diameters measured by SANS are smaller than observed by TEM, which may indicate SANS detecting a protofilament structure not observable on the length scales probed by TEM. 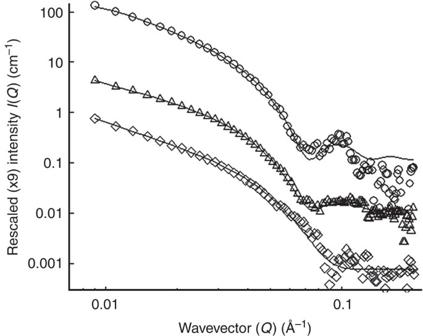Figure 5: Small angle neutron scattering (SANS) data. SANS data for (○)1alone, ()2alone and (Δ)1and2. Figure 5: Small angle neutron scattering (SANS) data. SANS data for ( ○ ) 1 alone, ( ) 2 alone and (Δ) 1 and 2 . Full size image For mixed gels, the scattering was more complex, demonstrating characteristic peaks associated with both pure 1 and pure 2 (slow decay at low Q indicative of 2 , and the precipitous feature of 1 around Q max ≈ 0.08 Å −1 ). Both the mixed sample and pure 1 show a weak peak around Q max ≈ 0.10 Å −1 (63 Å) indicating that both contain some degree of core-shell morphology. However, a comparison of the scattering from pure and mixed gels alone could not distinguish between coexisting homomolecular assemblies and coassembled average structures. To clarify this distinction, we prepared an analogue of 2 with a deuterated naphthalene ring ( d-2 ), which will greatly reduce the contribution of 2 to the scattering. The fit to the SANS data from gels containing pure d-2 was in close agreement with that of 2 , albeit with significantly weaker scattering as expected, indicating that the assembly of 2 is unaffected by deuteration ( Supplementary Figs S5 and S6 ). We then examined mixed systems of 1 and d-2 . Here if the system were truly mixed, we would expect an overall decrease in scattering when using d-2 as compared with 2 . For a self-sorted system, we would expect that the scattering would more resemble that of 1 alone, as the scattering from d-2 is reduced relative to 2 . This latter case is indeed what we see: comparing scattering from the mixture of 1 and 2 with that from either 1 or d-2 shows a relative increase in the contribution of the feature at 0.10 Å −1 ; that is, the scattering from a mixture of 1 and d-2 resembles most strongly the scattering from 1 ( Supplementary Fig. S7 ). Hence, the SANS data is consistent with a self-sorted system being formed rather than an average structure. Fibre X-ray diffraction proves self-sorting To prove definitively the self-sorting of 1 and 2 at the assembled molecular level, we used fibre X-ray diffraction (fXRD) of the gel phase as shown in Fig. 6 . We have used this technique previously to examine gels formed from both 1 (ref. 13 ) and 2 (ref. 23 ) in single-component systems, and have shown that it is appropriate for studying hydrated gel phases [23] . The diffraction from 1 differs significantly to that from 2 ,producing a characteristic and reproducible signature for each individual system. In confirmation of self-sorting, the fXRD pattern of the two-component system was found to match an overlay of the scattering signatures expected from individual ‘pure’ gels ( Fig. 6b ). Importantly, the signal positions arising from the lattice structures of the individual systems are preserved in the mixed gel. Had coassembly occurred, a disruption of the individual native lattice structures or the formation of a new unique structure would be expected. A slight difference is observed in the relative intensity of the expected equatorial signal at ~20 Å, arising from 1 , though this can be attributable to differing fibre packing arrangements influenced by the presence of 2 . Therefore, we conclude that the single-component system structures are unchanged, indicating that self-sorting has occurred. This is remarkable when one considers the structural similarity between the two gelator precursors, and the identical chirality of both molecules: indeed, these two parameters are most often used to define and to design self-sorted systems [1] , [2] , [11] . We note that it is possible that a block-like structure has been adopted, whereby fibres formed from 2 nucleate from the ends of fibres of 1 . From the TEM data, this seems unlikely, but we cannot currently rule out this possibility. 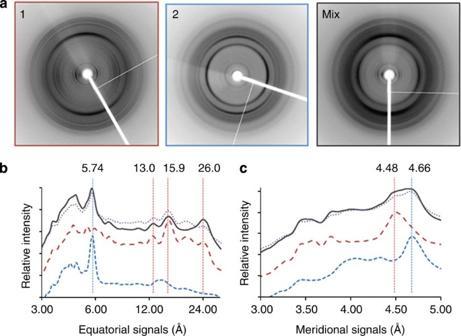Figure 6: fXRD data show self-sorting. (a) fXRD data for1alone (left),2alone (middle) and the two-component system (right). (b) Equatorial and (c) meridional intensities for (red, long dash)1, (blue, short dash)2and (black, solid) the two-component system. The calculated theoretical self-sorted combination (purple, dotted) of1and2is shown for reference. Significant matching peaks are labelled in Ångstroms and their origin coloured by respective systems as above. Equatorial signals are shown over a logarithmic scale for clarity. Figure 6: fXRD data show self-sorting. ( a ) fXRD data for 1 alone (left), 2 alone (middle) and the two-component system (right). ( b ) Equatorial and ( c ) meridional intensities for (red, long dash) 1 , (blue, short dash) 2 and (black, solid) the two-component system. The calculated theoretical self-sorted combination (purple, dotted) of 1 and 2 is shown for reference. Significant matching peaks are labelled in Ångstroms and their origin coloured by respective systems as above. Equatorial signals are shown over a logarithmic scale for clarity. Full size image Shape, size and chirality have all been used to direct self-sorting previously, coupled with thermal gelation methods. Our results show that pH can also be used to bring about self-sorting, even for gelators with very similar structures. Self-sorting processes have been reported to be either under thermodynamic or kinetic control [1] , [2] . In the thermodynamic case, the system is at its most stable when self-sorted [26] . Kinetic self-sorting, on the other hand, relies on a fast formation to ensure that a self-sorted local minimum, as opposed to the thermodynamic minimum, is reached [27] . In the case of gelators, it is not at all clear that the gel state represents the thermodynamic minimum. Indeed, we have shown recently that under some conditions, crystallization of 2 from the gel phase occurs, which is presumably a lower energy state [23] . Nevertheless, the pH triggered methodology presented here utilizes kinetic control to ensure self-sorting and offers an interesting and useful alternative concept to the routes currently reported. This chemically triggered route may allow us to access metastable materials and phases that are simply inaccessible via conventional routes because we temporally separate the individual assembly processes, based on the underlying chemistry that promotes molecular aggregation. In terms of the relative importance of the kinetic and thermodynamic aspects, we tested the process to the extreme by using a mineral acid, hydrochloric acid, to adjust the pH, as opposed to GdL. This removes the buffering effect from the p K a of the components and is expected to magnify kinetic effects. Indeed, as we reported elsewhere [16] , the use of a mineral acid to adjust the pH results in less uniform gels on a macroscopic level. The fXRD of this gel shows that the alignment is lost. However, the fXRD data shows that the gel is still inherently self-sorted, with reflections attributable to 1 and 2 clearly being seen ( Supplementary Fig. S8 ). This implies that the self-sorting is thermodynamically preferred as opposed to being solely a result of the kinetic process. It is difficult to deconvolute whether the difference in p K a or molecular structure is the key feature leading to this thermodynamic preference for self-sorting. The difference in p K a is driven by the difference in hydrophobicity for these molecules. Hence, to adjust the p K a , it is necessary to adjust the molecular structure. It is clear, nonethless, that the kinetic process allows a high degree of control over the assembly process, although we note also that our GdL route may allow access to materials that do not thermodynamically self-sort in this way in response to mineral acid. This pH-based system offers several key advantages. The pH at which the assembly of each component occurs is determined by the apparent p K a of the gelator. This correlates with the overall hydrophobicity of the gelator, which could potentially be specified as required by tuning of the molecular structure. Uniquely, this method allows the order of assembly to be predefined. Further, this method allows control over the self-sorting: it is possible to alter the rate at which self-sorting occurs, as well as affecting whether one or both gelators self-assemble. We suggest that this could be expanded to more complex, information-rich systems, involving a greater numbers of gelators. This method is not restricted to functionalised dipeptide gelators; a number of other molecules form gels via a decrease in pH and since our first report, using the GdL method [28] . Further, it is likely that this method will cause the microstructure to be affected in addition to the nanostructure by control over the rate of pH decrease. It may then be possible to further react or covalently cross-link one of the gelators to lock in these microstructures as shown elsewhere [29] . We envisage that this methodology will be suitable for the generation of new p-n bulk heterojunctions along with other high value applications. Synthetic details See Supplementary Methods for full synthetic procedures. The deuterated analogue of 2 ( d-2 ) was synthesized via a multistep procedure and the intermediate deuterated complexes S1 , S2 , S3 , S4 and S5 were isolated and characterized, see Supplementary Methods . NMR experiment to monitor self-sorting Dipeptide 1 and 2 (25.0 mg of each) were suspended in D 2 O (5 ml). An equimolar quantity of NaOD (1 M, aq) was added, and the solution was gently stirred for 30 min until a clear solution was formed. The pD of this solution was measured to be 10.5. Ethanol (10 μl) was added as internal reference. 1 H NMR spectra were recorded at 400.13 MHz using a Bruker Avance 400 NMR spectrometer. To prepare hydrogels, solutions were added to measured quantities of GdL according to the requirements of final pH ( Supplementary Table S1 ). The sample was then loaded immediately into the spectrometer. A spectrum was collected every 5 min. Data was analysed using Topspin. Fibre X-ray diffraction 1 and 2 were dissolved in D 2 O with equimolar amounts of NaOD. The final pD of the solutions were measured to be 10.5 after fine adjustment of the pD with dilute NaOD. Individual gelation of the systems was initiated by thorough but gentle mixing of GdL with a solution containing either 1 or 2 . Mixed gels containing both systems were prepared by mixing GdL with a solution of 1 and 2 . Fibres were aligned from these gelating solutions by in situ methods as described previously [13] , [23] . Diffraction data was collected using a Rigaku 007HF Cu Kα (λ 1.5419 Å) rotating anode generator with VariMax-HF mirrors and Saturn 944+ CCD (charge-coupled device) detector. Exposure times were 20 s at specimen to detector distances of 50 mm. Diffraction patterns were converted to .tiff files using mosflm and processed using CLEARER [30] . Diffraction signal intensity traces were produced by converting diffraction signals as a function of pixels to Ångstroms using Bragg’s law. The graphical theoretical combination in Fig. 6b was calculated by summation of the single-component diffraction traces. Additional techniques The SANS, TEM, rheology and SEM experimental details are described in the Supplementary Methods . How to cite this article: Morris, K. L. et al . Chemically programmed self-sorting of gelator networks. Nat. Commun. 4:1480 doi: 10.1038/ncomms2499 (2013).